Skp2–MacroH2A1–CDK8 axis orchestrates G2/M transition and tumorigenesis Understanding the mechanism by which cell growth, migration, polyploidy, and tumorigenesis are regulated may provide important therapeutic strategies for cancer therapy. Here we identify the Skp2–macroH2A1 (mH2A1)–cyclin-dependent kinase 8 (CDK8) axis as a critical pathway for these processes, and deregulation of this pathway is associated with human breast cancer progression and patient survival outcome. We showed that mH2A1 is a new substrate of Skp2 SCF complex whose degradation by Skp2 promotes CDK8 gene and protein expression. Strikingly, breast tumour suppression on Skp2 deficiency can be rescued by mH2A1 knockdown or CDK8 restoration using mouse tumour models. We further show that CDK8 regulates p27 protein expression by facilitating Skp2-mediated p27 ubiquitination and degradation. Our study establishes a critical role of Skp2–mH2A1–CDK8 axis in breast cancer development and targeting this pathway offers a promising strategy for breast cancer therapy. Maintaining genomic integration and proper cell cycle entry is a critical failsafe mechanism for preventing cancer initiation and progression [1] , [2] . Cancer cells often display aberrant cell cycle and higher degree of aneuploidy and/or polyploidy [3] . How these events occur during the cancer progression remains largely unclear. Understanding the regulatory mechanism that orchestrates these processes may provide new therapeutic strategies for cancer prevention and treatment. Skp2 is an F-box protein that forms an SCF complex with Skp1 and Cullin-1 to constitute E3 ligase and plays a critical role in cell cycle regulation, maintenance of genomic integrity and cancer development [4] , [5] , [6] , [7] . As a consequence, primary Skp2 -deficient mouse embryonic fibroblasts (MEFs) display upregulated p27 expression and higher percentage of G2/M phase and polyploidy. Notably, loss of p27 can revere G2/M arrest and polyploidy in primary Skp2 -deficient MEFs, suggesting that p27 is a relevant substrate for Skp2 and is responsible for G2/M arrest and polyploidy on Skp2 deficiency [8] , [9] , [10] , [11] . However, recent study reveals that p27 silencing does not rescue G2/M arrest and polyploidy in p53-mutant melanoma cells on Skp2 knockdown [12] . Accordingly, these results imply that in addition to p27, Skp2 may also impact other pathways to orchestrate G2/M arrest and polyploidy under distinct genetic contexts. Using affinity purification in conjunction with mass spectrometry analysis, we identified MacroH2A1 (mH2A1) also known as H2AFY as a novel binding partner for Skp2. mH2A is an epigenetic factor that primarily localizes in the heterochromatin and cooperates with HP1 to induce transcriptional repression, thereby leading to X chromosome inactivation [13] . mH2A consists of mH2A1 (mH2A1.1 and mH2A1.2) and mH2A2 isoforms, which may share similar functions [14] , [15] , [16] . A recent study revealed that mH2A1 is a potential tumour suppressor whose expression is lost in advanced melanoma due to its promoter hypermethylation, and that its overexpression leads to the suppression of melanoma development [17] . Although the promoter hypermethylation of mH2A1 is proposed as a potential mechanism by which mH2A1 expression is lost in melanoma, how its activity and protein stability are regulated remain completely puzzled. In this study, we unravel that Skp2 is a novel E3 ligase for mH2A1 and triggers mH2A1 ubiquitination and degradation, in turn leading to cyclin-dependent kinase 8 (CDK8) gene expression. Notably, we find that upregulation of mH2A1 and subsequent CDK8 downregulation contributes to growth defect, G2/M arrest, polyploidy and tumour suppression on Skp2 loss. Finally, we show that CDK8 is a novel regulator of p27 by facilitating Skp2-mediated ubiquitination and degradation of p27. Our study not only reveals novel insights into how mH2A1 stability is regulated, but also establishes a new role of mH2A1-CDK8 in Skp2-mediated cell cycle regulation, genomic stability and tumorigenesis. Skp2 interacts with mH2A1 To define the novel mechanism by which Skp2 regulates G2/M arrest and polyploidy, we performed a systematic approach to identify novel Skp2 binding partners. To this end, we generated 293T cells stably overexpressed with Xpress-Skp2 (XP-Skp2), and the total cell lyates from these cells were immunoprecipitated with Xpress antibody to pull down XP-Skp2 and Skp2 interacting proteins were identified by mass spectrometry analysis. Using this approach, we were able to obtain several peptides existed in Skp2 immunocomplex that correspond to mH2A1 ( Fig. 1a ). These peptides can be found in mH2A1.1 and mH2A1.2. mH2A is an epigenetic factor that regulates X chromosome inactivation and serves as a potential tumour suppressor for melanoma development [13] , [17] . 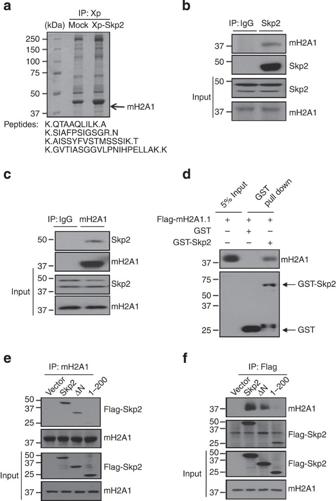Figure 1: Skp2 interacts with mH2A1. (a) Lysates from 293T stably transfected with vector or Xpress-Skp2 (XP-Skp2) were immunoprecipitated with XP antibody and subjected to mass spectrometry analysis. Histone variant mH2A1 was identified as a novel binding partner for Skp2. (b,c) 293T cells were harvested for immunoprecipitation with Skp2 antibody (b) or mH2A1 antibody (c), followed by immunoblotting. (d)In vitroGST pull-down assay using recombinant GST, GST–Skp2 proteins purified from bacteria andin vitrotranslated Flag–mH2A1.1. 5% of input was loaded in this assay. (e,f) 293T cells were transfected with indicated plasmids and harvested for immunoprecipitation assay. Figure 1: Skp2 interacts with mH2A1. ( a ) Lysates from 293T stably transfected with vector or Xpress-Skp2 (XP-Skp2) were immunoprecipitated with XP antibody and subjected to mass spectrometry analysis. Histone variant mH2A1 was identified as a novel binding partner for Skp2. ( b , c ) 293T cells were harvested for immunoprecipitation with Skp2 antibody ( b ) or mH2A1 antibody ( c ), followed by immunoblotting. ( d ) In vitro GST pull-down assay using recombinant GST, GST–Skp2 proteins purified from bacteria and in vitro translated Flag–mH2A1.1. 5% of input was loaded in this assay. ( e , f ) 293T cells were transfected with indicated plasmids and harvested for immunoprecipitation assay. Full size image To validate the interaction between Skp2 and mH2A1, we performed the reciprocal co-immunoprecipitation (Co-IP) experiments and found that endogenous Skp2 interacted with endogenous mH2A1 ( Fig. 1b,c ). In vitro glutathione S-transferase (GST) pull-down assay revealed that Skp2 could interact with mH2A1 ( Fig. 1d ). We further demonstrated that C-terminal of Skp2 (amino acids 201–424) and N-terminal region of mH2A1 are required for the interaction between Skp2 and mH2A1 by using Co-IP assays ( Fig. 1e,f and Supplementary Fig.1a ). Immunofluorescence assay further revealed that Skp2 was co-localized with mH2A1.1 and mH2A1.2 in nucleus in MDA-MB-231 breast cancer cells ( Supplementary Fig. 1b ). Skp2 SCF directly triggers ubiquitination and degradation of its protein substrates. Since Skp2 normally binds to its protein substrates though Skp2 C-terminal LRR (leucine-rich repeat) domain, it is highly possible that mH2A1 is a novel Skp2 substrate. To test this hypothesis, we conducted in vivo ubiquitination assay to determine whether Skp2 promotes mH2A1 ubiquitination. Notably, overexpression of Skp2, but not of E3 ligase-dead Skp2-LRR mutant, promoted ubiquitination of mH2A1.1 in the presence of proteosome inhibitor MG132 ( Fig. 2a ), suggesting that Skp2 SCF is likely an E3 ligase for mH2A1. Similar results were also obtained for mH2A1.2 ( Supplementary Fig. 1c ). To corroborate the notion that Skp2 SCF is a direct E3 ligase for mH2A1, we performed in vitro ubiquitination assay and found that Skp2 SCF could induce mH2A1 ubiquitination in vitro ( Fig. 2b ). Notably, we found that ubiquitination of mH2A1.1 and mH2A1.2 was profoundly reduced on Skp2 knockdown ( Fig. 2c and Supplementary Fig. 1d ), suggesting that Skp2 is required for ubiquitination of mH2A1.1 and mH2A1.2. We further demonstrated that Skp2 triggered K48-linked ubiquitination of mH2A1.1, while it induced K63-linked ubiquitination of Akt ( Fig. 2d ). Accordingly, these results suggest that mH2A1 is a novel substrate for Skp2. 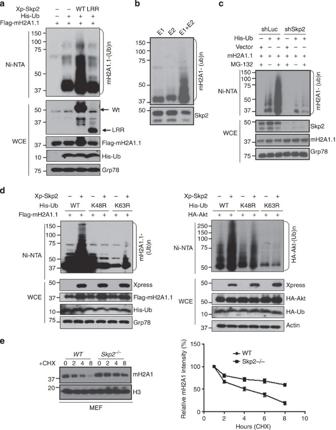Figure 2: Skp2 SCF is a direct E3 ligase for mH2A1 and triggers ubiquitination and degradation of mH2A1. (a)In vivoubiquitination assay from 293T cells transfected with indicated plasmids. (b) Flag–Skp2 proteins isolated 293T cells transfected with Flag–Skp2 were incubated with ATP, E1, E2 along with mH2A1 proteins isolated from 293T cells forin vitroubiquitination assay. (c) 293T cells stably expressing luciferase shRNA (shLuc) or Skp2 shRNA (shSkp2) were transfected with the indicated plasmids and harvested forin vivoubiquitination assay. (d)In vivoubiquitination assay of 293T cells transfected with His-Ubiquitin (His-Ub), His-Ub K48R or His-Ub K63R along with other constructs. (e) PrimaryWTandSkp2−/−MEFs were treated with cycloheximide for the indicated times and harvested for immunoblotting analysis. A representative blot and quantification from there independent experiments were shown. CHX, cycloheximide; Ni-NTA, nickel bead pulldown; WCE, whole-cell extracts. Figure 2: Skp2 SCF is a direct E3 ligase for mH2A1 and triggers ubiquitination and degradation of mH2A1. ( a ) In vivo ubiquitination assay from 293T cells transfected with indicated plasmids. ( b ) Flag–Skp2 proteins isolated 293T cells transfected with Flag–Skp2 were incubated with ATP, E1, E2 along with mH2A1 proteins isolated from 293T cells for in vitro ubiquitination assay. ( c ) 293T cells stably expressing luciferase shRNA (shLuc) or Skp2 shRNA (shSkp2) were transfected with the indicated plasmids and harvested for in vivo ubiquitination assay. ( d ) In vivo ubiquitination assay of 293T cells transfected with His-Ubiquitin (His-Ub), His-Ub K48R or His-Ub K63R along with other constructs. ( e ) Primary WT and Skp2 −/− MEFs were treated with cycloheximide for the indicated times and harvested for immunoblotting analysis. A representative blot and quantification from there independent experiments were shown. CHX, cycloheximide; Ni-NTA, nickel bead pulldown; WCE, whole-cell extracts. Full size image K48-linked ubiquitination is linked to proteosome-dependent degradation [18] . The finding that Skp2 promotes K48-linked ubiquitination of mH2A1 in a proteosome-dependent manner suggests that Skp2 may regulate mH2A1 protein level and stability. Consistent with this notion, we found that mH2A1 protein level was upregulated in primary Skp2 −/− MEFs compared with wild-type ( WT ) MEFs ( Supplementary Fig. 1e ). We also confirm this result by demonstrating that Skp2 knockdown in various cancer cells induced mH2A1 protein expression ( Supplementary Fig. 2a,b ), correlated with a reduction in ubiquitination of mH2A1.1 and mH2A1.2 on Skp2 knockdown ( Fig. 1c and Supplementary Fig. 1d ). In accordance with its protein expression, mH2A1 protein stability was also higher in Skp2 −/− MEFs and Skp2 knockdown breast cancer cells ( Fig. 2e and Supplementary Fig. 3a ). Moreover, we showed that Skp2 overexpression in breast cancer cells reduced mH2A1 protein levels ( Supplementary Fig. 2c ) and protein stability ( Supplementary Fig. 3b ). Our results therefore suggest that Skp2 SCF is the E3 ligase for mH2A1, which promotes mH2A1 ubiquitination and degradation. mH2A1 regulates G2/M arrest and polyploidy on Skp2 loss Primary Skp2 −/− MEFs display profound reduction in cell proliferation and migration, but higher percentage of G2/M phase and polyploidy [11] , [19] , [20] . The finding that mH2A1 protein expression is induced in Skp2 −/− MEFs prompted us to test whether mH2A1 overexpression recapitulates the phenotypes in Skp2 -deficient cells. Indeed, we found that mH2A1.1 overexpression induced growth arrest, G2/M arrest and polyploidy, mirroring the phenotypes on Skp2 deficiency in MEFs ( Fig. 3a–d ). We next determined whether mH2A1 upregulation is responsible for these phenotypes observed in Skp2 −/− MEFs. To achieve this goal, we knocked down mH2A1 in Skp2 −/− MEFs ( Fig. 4a ) and determined whether the phenotypes from Skp2 −/− MEFs are rescued. FACS analysis revealed that while primary Skp2 −/− MEFs exhibited much higher percentage of G2/M phase and polyploidy compared with WT MEFs, mH2A1 knockdown could significantly rescue these phenotypes ( Fig. 4b–d ), suggesting that mH2A1 upregulation contributes to G2/M arrest and polyploidy in Skp2 −/− MEFs. 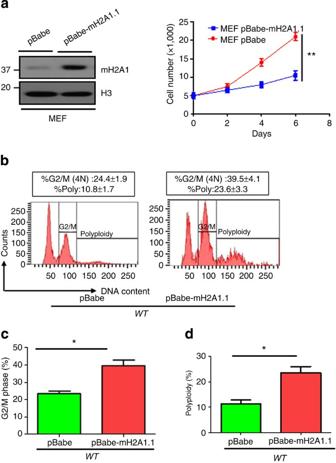Figure 3: mH2A1.1 overexpression in primary MEFs triggers cell growth arrest and polyploidy. (a) Primary MEFs were infected with pBabe or pBabe–mH2A1.1 lentiviral RNAs, selected and harvested for immunoblotting (left panel). These cells were plated in 24-well plated for cell growth assay using direct cell counting (right panel). (b) Flow cytometry analysis of DNA content in primary MEFs stably expressing pBabe or pBabe–mH2A1.1. (c) G2/M phase was determined by flow cytometry analysis of primaryWTMEFs with stably expressing pBabe or pBabe–mH2A1.1. The quantified results are presented as mean±s.d. (d) Polyploidy of primaryWTandSkp2−/−MEFs with stably expressing pBabe or pBabe–mH2A1.1. The quantified results are presented as means±s.d. Error bars indicate s.e.m. Data represent mean values of three independent experiments. Student’st-test used: *P<0.05; **P<0.01). Figure 3: mH2A1.1 overexpression in primary MEFs triggers cell growth arrest and polyploidy. ( a ) Primary MEFs were infected with pBabe or pBabe–mH2A1.1 lentiviral RNAs, selected and harvested for immunoblotting (left panel). These cells were plated in 24-well plated for cell growth assay using direct cell counting (right panel). ( b ) Flow cytometry analysis of DNA content in primary MEFs stably expressing pBabe or pBabe–mH2A1.1. ( c ) G2/M phase was determined by flow cytometry analysis of primary WT MEFs with stably expressing pBabe or pBabe–mH2A1.1. The quantified results are presented as mean±s.d. ( d ) Polyploidy of primary WT and Skp2 −/− MEFs with stably expressing pBabe or pBabe–mH2A1.1. The quantified results are presented as means±s.d. Error bars indicate s.e.m. Data represent mean values of three independent experiments. Student’s t -test used: * P <0.05; ** P <0.01). 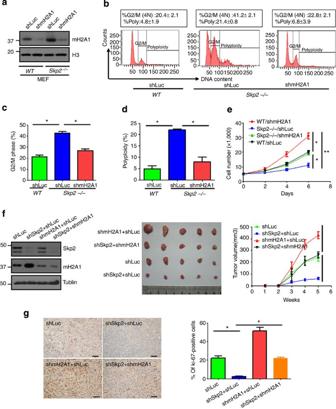Figure 4: mH2A1 deficiency rescues cell growth arrest and polyploidy onSkp2loss. (a) PrimaryWTandSkp2−/−MEFs were infected with luciferase shRNAs (shLuc) or mH2A1 shRNAs (shmH2A1), selected and harvested for immunoblotting. (b) Flow cytometry analysis of DNA content inWTandSkp2−/−MEFs with Luc or mH2A1 knockdown. (c) G2/M phase was determined by flow cytometry analysis of primaryWTandSkp2−/−MEFs with stably expressing shLuc or shmH2A1. (d) Polyploidy of primaryWTandSkp2−/−MEFs with stably expressing shLuc or shmH2A1. (e) Cell growth assay by direct cell counting ofWTandSkp2−/−MEFs with Luc or mH2A1 knockdown. (f) MDA-MB-231 cells infected with various shRNAs were subcutaneously injected into nude mice (n=5 for each group). Tumour size was monitored and calculated by caliper for up to 5 weeks (see Methods). The cell lysates from tumour cells were subjected to immunoblotting (left panel). A photo of five tumours aligned together were presented (middle panel). The results were calculated as mean values±s.d. (g) MDA-MB-231 cells infected with various shRNAs were subcutaneously injected into nude mice, and breast tumours were harvested from nude mice at week 5 for Ki-67 staining by IHC and quantitated (Scale bars, 50 μm). Error bars indicate s.e.m. Data represent mean values of three independent experiments. Student'st-test used: *P<0.05; **P<0.01). Full size image Figure 4: mH2A1 deficiency rescues cell growth arrest and polyploidy on Skp2 loss. ( a ) Primary WT and Skp2 −/− MEFs were infected with luciferase shRNAs (shLuc) or mH2A1 shRNAs (shmH2A1), selected and harvested for immunoblotting. ( b ) Flow cytometry analysis of DNA content in WT and Skp2 −/− MEFs with Luc or mH2A1 knockdown. ( c ) G2/M phase was determined by flow cytometry analysis of primary WT and Skp2 −/− MEFs with stably expressing shLuc or shmH2A1. ( d ) Polyploidy of primary WT and Skp2 −/− MEFs with stably expressing shLuc or shmH2A1. ( e ) Cell growth assay by direct cell counting of WT and Skp2 −/− MEFs with Luc or mH2A1 knockdown. ( f ) MDA-MB-231 cells infected with various shRNAs were subcutaneously injected into nude mice ( n =5 for each group). Tumour size was monitored and calculated by caliper for up to 5 weeks (see Methods). The cell lysates from tumour cells were subjected to immunoblotting (left panel). A photo of five tumours aligned together were presented (middle panel). The results were calculated as mean values±s.d. ( g ) MDA-MB-231 cells infected with various shRNAs were subcutaneously injected into nude mice, and breast tumours were harvested from nude mice at week 5 for Ki-67 staining by IHC and quantitated (Scale bars, 50 μm). Error bars indicate s.e.m. Data represent mean values of three independent experiments. Student's t -test used: * P <0.05; ** P <0.01). Full size image Notably, we found that growth defect in Skp2 −/− MEFs could be partially rescued by mH2A1 knockdown ( Fig. 4e ). Similarly, mH2A1 knockdown also rescued the growth defect of two breast cancer cell lines with Skp2 silencing ( Supplementary Fig. 4a,b ), as determined by cell proliferation and colony forming assays ( Supplementary Fig. 4c ). Moreover, we found that cell migration defect on Skp2 knockdown in breast cancer cells could be also rescued by mH2A1 knockdown ( Supplementary Fig. 4d ). mH2A1 mediates tumour suppression on Skp2 knockdown Recent studies reveal that Skp2 overexpression promotes cancer development, but its deficiency leads to tumour suppression [4] , [5] , [6] , [19] , [20] . We next sought to determine whether mH2A1 upregulation accounts for breast tumour suppression on Skp2 silencing. Remarkably, while Skp2 silencing markedly reduced breast cancer development, mH2A1 knockdown reversed such tumour suppressive effect ( Fig. 4f ). Consistent with results in cell models, breast tumour with Skp2 deficiency also displayed enhanced mH2A1 protein expression ( Supplementary Fig. 4e ). It should be noted that mH2A1 knockdown promoted breast cancer development ( Fig. 4f ). The immunohistochemistry (IHC) staining in breast tumours revealed that Skp2 knockdown reduced breast cancer cell proliferation in vivo , as determined by Ki-67 staining, and such suppression effect could be rescued by mH2A1 knockdown ( Fig. 4g ). However, there was no obvious difference in apoptosis between Skp2 knockdown versus both Skp2 and mHA1 knockdown groups ( Supplementary Fig. 4f ). Accordingly, these results suggest that mH2A1 induction serves as a tumour suppressive signal responsible for inhibition of cell growth, cell migration and breast cancer development on Skp2 deficiency. CDK8 restoration rescues the phenotypes on Skp2 loss To understand how Skp2-mediated mH2A1 ubiquitination and degradation regulates G2/M arrest, polyploidy, cell migration and tumorigenesis, we performed the systematically non-biased microarray analysis in primary WT and Skp2 -deficient cells. We found that around 3,000 genes were upregulated, but 4,000 genes were downregulated on Skp2 deficiency (data were deposited to GEO as GSE23064). As mH2A1 is a transcription repressor, upregulation of mH2A1 observed in Skp2 deficiency cells should lead to gene repression. We therefore focused on the genes downregulated in Skp2 -deficient cells. Among those genes downregulated on Skp2 deficiency, we found that CDK8 (cyclin-dependent kinase 8) was the gene whose messenger RNA (mRNA) expression was profoundly reduced in Skp2 -deficient cells ( Supplementary Table 1 ). We selected CDK8 for further study because of its important role in cancer regulation [21] , [22] . CDK8 is a component of the mediator complex consisting of CDK8, Cyclin C, Med12 and Med13, which can serve as either a transcription activator or repressor dependently of distinct promoters of its target genes. Interestingly, CDK8 can also indirectly regulate gene expression through directly phosphorylating its protein substrates, such as receptor activated Smads and E2F1, and likely independently of mediator complex formation [23] , [24] , [25] . CDK8 displays an oncogenic activity in melanoma and colon cancer [21] , [22] . To confirm our microarray results, we performed real-time PCR analysis to determine the mRNA level of CDK8 expression in various cancer cells on Skp2 overexpression or knockdown. Consistently, we found that Skp2 overexpression promoted mRNA level of CDK8, while its knockdown reduced it ( Fig. 5a ). In accordance with the real-time PCR analysis, Western blot analysis revealed that Skp2-overexpressed breast cancer cells displayed higher CDK8 protein expression, whereas Skp2 knockdown cells exhibited less CDK8 protein expression ( Fig. 5b,c ). Accordingly, Skp2 is therefore a novel upstream regulator for CDK8 gene and protein expression. 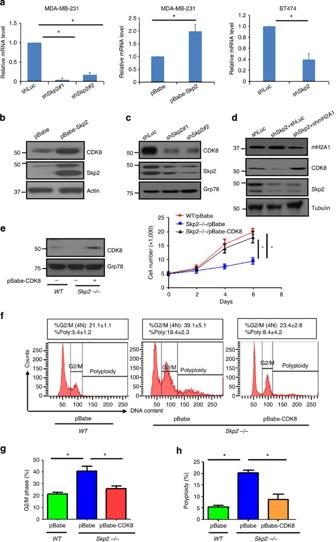Figure 5: CDK8 is a downstream effector responsible for Skp2-mediated cell growth, G2/M and polyploidy. (a) The mRNA levels of CDK8 were measured by real-time PCR in MDA-MB-231 and BT474 cells with Luc or Skp2 knockdown (n=3). (b–d) Immunoblotting of MDA-MB-231 cells infected with pBabe or pBabe–Skp2 (b), infected with Luc or Skp2 shRNAs (c) or infected with Luc shRNAs, Skp2 shRNAs or Skp2 plus mH2A1 shRNAs (d). (e) Immunoblotting assay (left panel) and cell growth assay by direct cell counting (right panel) of primaryWTandSkp2−/−MEFs with stably expressing pBabe or pBabe–CDK8. (f) Flow cytometry analysis of DNA content in primaryWTandSkp2−/−MEFs with stably expressing pBabe or pBabe–CDK8. (g) G2/M phase was determined by Flow cytometry analysis of primaryWTMEFs with stably expressing pBabe or pBabe–CDK8. (h) Polyploidy of primaryWTandSkp2−/−MEFs with stably expressing pBabe or pBabe–CDK8. (Error bars indicate s.e.m. Data represent mean values of three independent experiments. Student’st-test used: *P<0.05). Figure 5: CDK8 is a downstream effector responsible for Skp2-mediated cell growth, G2/M and polyploidy. ( a ) The mRNA levels of CDK8 were measured by real-time PCR in MDA-MB-231 and BT474 cells with Luc or Skp2 knockdown ( n =3). ( b – d ) Immunoblotting of MDA-MB-231 cells infected with pBabe or pBabe–Skp2 ( b ), infected with Luc or Skp2 shRNAs ( c ) or infected with Luc shRNAs, Skp2 shRNAs or Skp2 plus mH2A1 shRNAs ( d ). ( e ) Immunoblotting assay (left panel) and cell growth assay by direct cell counting (right panel) of primary WT and Skp2 −/− MEFs with stably expressing pBabe or pBabe–CDK8. ( f ) Flow cytometry analysis of DNA content in primary WT and Skp2 −/− MEFs with stably expressing pBabe or pBabe–CDK8. ( g ) G2/M phase was determined by Flow cytometry analysis of primary WT MEFs with stably expressing pBabe or pBabe–CDK8. ( h ) Polyploidy of primary WT and Skp2 −/− MEFs with stably expressing pBabe or pBabe–CDK8. (Error bars indicate s.e.m. Data represent mean values of three independent experiments. Student’s t -test used: * P <0.05). Full size image CDK8 gene expression was negatively regulated by mH2A [17] . Given Skp2 promotes mH2A1 ubiquitination and degradation, it is highly possible that Skp2 regulates CDK8 expression by promoting mH2A1 degradation. To test this hypothesis, we silenced mH2A1 expression in the context of Skp2 knockdown to assess CDK8 expression. As expected, while Skp2 knockdown markedly reduced CDK8 protein expression, mH2A1 silencing rescued this effect ( Fig. 5d ), suggesting that Skp2 induces CDK8 expression acting through mH2A1 degradation. We next investigated whether CDK8 is a critical downstream player that executes Skp2-medaied G2/M transition, polyploidy and cell proliferation. Notably, we found that CDK8 restoration partially rescued defect in cell growth, G2/M arrest and polyploidy observed in Skp2 −/− MEFs ( Fig. 5e–h ). It should be noted that the effect of Skp2, mH2A1 and CDK8 on G2/M arrest and polyploidy can be seen in primary MEFs, but not in breast cancer cells such as MDA-MB-231 cells. Since MDA-MB-231 display diverse genetic alterations like p53 mutations, it is likely that some of genetic alterations may affect the effect of Skp2, mH2A1 and CDK8 on G2/M arrest and polyploidy. Altogether, these results suggest that Skp2 promotes mH2A1 degradation and CDK8 expression, in turn regulating cell growth, G2/M transition and polyploidy in primary MEFs. CDK8 rescues breast cancer development on Skp2 loss To understand whether CDK8-mediated Skp2’s oncogenic activity, we restored CDK8 expression in Skp2 knockdown breast cancer cells for cell proliferation and cell migration assays. Strikingly, while Skp2 knockdown inhibited breast cancer cell proliferation and migration, restoration of CDK8 in Skp2 knockdown cancer cells rescued these defects ( Supplementary Fig. 5a,b ), to the extent similar to that regulated by mH2A1 knockdown ( Supplementary Fig. 4a ). As CDK8 rescues defect in breast cancer cell growth on Skp2 knockdown, we examined whether CDK8 may regulate cell cycle profile in breast cancer cells. FACS (Fluorescence-activated cell sorting) analysis revealed that CDK8 knockdown did not obviously affect cell cycle phases ( Supplementary Fig. 5c ). Strikingly, we found that CDK8 restoration rescued the defect in breast cancer development on Skp2 knockdown ( Fig. 6a ). Skp2 knockdown reduced breast cancer cell proliferation in vivo and such suppression effect could be rescued by CDK8 restoration ( Supplementary Fig. 5d ). However, no obvious difference in apoptosis was observed between groups. Altogether, these results suggest that Skp2 promotes CDK8 expression to regulate cancer cell growth, migration and breast cancer development. 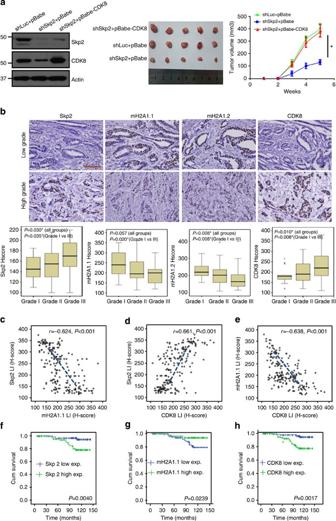Figure 6: CDK8 restoration recues the defect in tumorigenesis on Skp2 loss, and Skp2 expression inversely correlated with mH2A1, but positively correlated with CDK8 expression in human breast cancer samples. (a) Tumour volume (mm3) post-subcutaneous injections of MDA-MB-231 cells; *P<0.05 (n=5 mice per group). MDA-MB-231 cells silenced with control, Skp2 shRNAs or Skp2 shRNAs plus CDK8 overexpression were injected into nude mice (n=5 for each group) and followed up for tumorigenesis (see Methods). The lysate of tumour cells were subjected to immunoblotting (left panel). A photo of five tumours aligned together were presented (middle panel). The results were calculated as mean values±s.d. *P<0.05, **P<0.01 using Student’st-test (right panel). (b) Histological analysis of Skp2, mH2A1.1, mH2A1.2 and CDK8 expressions in patients with low or high grade of breast invasive ductal carcinoma. Scale bar, 200 μm. (c–e) Skp2 expression negatively correlated with mH2A1.1 (r=−0.624,P<0.001) (c), but positively associated with CDK8 (r=0.661,P<0.001) (d). mH2A1.1 negatively correlated with CDK8 expression (r=−0.638,P<0.001) (e). (f–h) Kaplan–Meier plot analysis of overall survival of 189 cases of breast invasive ductal carcinoma patients with low or high expression of Skp2 (f), mH2A1.1 (g) or CDK8 (h)Pvalue in all case is <0.01 by using Mann–WhitneyU-test. Figure 6: CDK8 restoration recues the defect in tumorigenesis on Skp2 loss, and Skp2 expression inversely correlated with mH2A1, but positively correlated with CDK8 expression in human breast cancer samples. ( a ) Tumour volume (mm 3 ) post-subcutaneous injections of MDA-MB-231 cells; * P <0.05 ( n =5 mice per group). MDA-MB-231 cells silenced with control, Skp2 shRNAs or Skp2 shRNAs plus CDK8 overexpression were injected into nude mice ( n =5 for each group) and followed up for tumorigenesis (see Methods). The lysate of tumour cells were subjected to immunoblotting (left panel). A photo of five tumours aligned together were presented (middle panel). The results were calculated as mean values±s.d. * P <0.05, ** P <0.01 using Student’s t -test (right panel). ( b ) Histological analysis of Skp2, mH2A1.1, mH2A1.2 and CDK8 expressions in patients with low or high grade of breast invasive ductal carcinoma. Scale bar, 200 μm. ( c – e ) Skp2 expression negatively correlated with mH2A1.1 ( r= −0.624, P <0.001) ( c ), but positively associated with CDK8 ( r= 0.661, P <0.001) ( d ). mH2A1.1 negatively correlated with CDK8 expression ( r= −0.638, P <0.001) ( e ). ( f – h ) Kaplan–Meier plot analysis of overall survival of 189 cases of breast invasive ductal carcinoma patients with low or high expression of Skp2 ( f ), mH2A1.1 ( g ) or CDK8 ( h ) P value in all case is <0.01 by using Mann–Whitney U -test. Full size image Skp2, mH2A1 and CDK8 expression in human breast cancer samples To understand the role of Skp2–mH2A1–CDK8 axis and their clinical correlations in human breast cancer, we performed IHC to determine the expression of these proteins in human breast cancer samples ( Fig. 6b ). In the 189 breast carcinomas, Skp2 overexpression was significantly associated with increments of primary tumour status (pT, P =0.030, Kruskal–Wallis H -test), nodal metastasis (pN, P <0.001, Mann–Whitney U -test) and stage ( P =0.001, Mann–Whitney U -test). mH2A1.1 (pN, P =0.017; stage, P =0.013, Mann–Whitney U -test) and mH2A1.2 (pT, P =0.028, Kruskal–Wallis H -test; and pN, P =0.001; stage, P =0.008, Mann–Whitney U -test) were negatively associated with adverse tumour features. Interestingly, CDK8 positively correlated with tumour status (pT, P =0.008, Kruskal–Wallis H -test), nodal metastasis (pN, P <0.001, Mann–Whitney U -test) and stage ( P <0.001, Mann–Whitney U -test) ( Table 1 ). As summarized in Table 2 , Fig. 6b–d and Supplementary Fig. 6a , Skp2 expression was negatively associated with mH2A1.1 ( r= −0.624, P <0.001, Pearson’s correlation coefficient test) and mH2A1.2 ( r= −0.578, P <0.001, Pearson’s correlation coefficient test) expression but positively associated with CDK8 ( r= 0.661, P <0.001, Pearson’s correlation coefficient test). Both mH2A1.1 and mH2A1.2 negatively correlated with CDK8 expression ( Fig. 6e , r= −0.638, P <0.001 and Supplementary Fig. 6b , r= −0.739, P <0.001, respectively, Pearson’s correlation coefficient test). Table 1 Associations between Skp2, MacroH2A1.1, MacroH2A1.2 and CDK8 expressions with important clinicopathologic variables. Full size table Table 2 Associations between Skp2, MacroH2A1.1, MacroH2A1.2 and CDK8 expressions in breast cancer. Full size table Notably, we found that all Skp2, mH2A1.1, mH2A1.2 and CDK8 expression significantly predicted disease-specific (DSS) and metastasis-free survival (MeFS) ( Table 3 ) , together with pT status, pN status and stage ( Fig. 6f–h , and Supplementary Fig. 6c–h ). In the multivariate analysis, only Skp2 overexpression remained prognostically significant for DSS. Of note, both Skp2 and CDK8 expression significantly predicted worse MeFS ( Table 4 ). These results along with the data from mouse tumour models suggest that Skp2–mH2A1–CDK8 axis serves as a critical signal for breast cancer development and represents an important biomarker for poor survival outcome of breast cancer patients. Table 3 Univariate log-rank analyses. Full size table Table 4 Multivariate survival analyses. Full size table CDK8 promotes p27 ubiquitination and degradation p27 is shown to be a critical substrate of Skp2 and is responsible for Skp2-mediated cell cycle progression, polyploidy and tumorigenesis. The finding that mH2A1–CDK8 axis also regulates Skp2-mediated cell cycle progression, polyploidy and tumorigenesis raises the possibility that CDK8 may function to cross-talk with p27. To test this hypothesis, we examined whether CDK8 regulates p27 expression. Although CDK8 knockdown failed to affect mRNA level of p27, it significantly induced p27 protein expression ( Supplementary Fig. 7b,e ). Conversely, CDK8 overexpression reduced p27 protein expression, but not p27 mRNA level ( Supplementary Fig. 7c–e ). Thus, CDK8 is a novel regulator for p27 protein expression. To gain insight into how CDK8 regulates p27 protein expression, we determined whether CDK8 may regulate ubiquitination and degradation of p27. Interestingly, we found that CDK8 overexpression promoted p27 ubiquitination ( Fig. 7a ), whereas CDK8 knockdown reduced it ( Fig. 7b ). As a consequence, CDK8 overexpression promoted p27 degradation, whereas CDK8 knockdown reduced it. Thus, CDK8 acts through p27 ubiquitnaiton and degradation to orchestrate p27 protein expression. 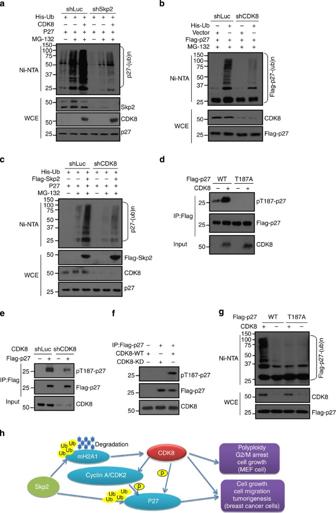Figure 7: CDK8 phosphorylate p27 at T187 and facilitates Skp2-mediated p27 ubiquitination and degradation. (a) 293T cells stably expressing luciferase shRNA (shLuc) or Skp2 shRNA (shSkp2) were transfected with the indicated plasmids and harvested forin vivoubiquitination assay. (b) 293T cells stably expressing luciferase shRNA (shLuc) or CDK8 shRNA (shCDK8) were transfected with the indicated plasmids and harvested forin vivoubiquitination assay. (c) 293T cells stably expressing luciferase shRNA (shLuc) or CDK8 shRNA (shCDK8) were transfected with the indicated plasmids and harvested forin vivoubiquitination assay. (d) Cell lysates from 293T cells transfected with vector or CDK8 along with WT Flag-p27 or Flag-p27-187A were immunoprecipitated with Flag antibody and subjected to the immunoblotting assay. p27 phosphorylation at T187 was detected by using an antibody against phosphorylated p27 at T187. (e) Cell lysates from Luc or CDK8 knockdown 293T cells transfected with vector or Flag-p27 were immunoprecipitated with Flag antibody and subjected to the immunoblotting assay. p27 phosphorylation at T187 was detected by using an antibody against phosphorylated p27 at T187. (f) CDK8 phosphorylates p27in vitro. Immunopurified Flag-p27 proteins were incubated with or without recombinant active CDK8 or CDK8-KD proteins and subjected to the immunoblotting assay. p27 phosphorylation at T187 was detected by using an antibody against phosphorylated p27 at T187. (g)In vivoubiquitination assay of 293T cells transfected with Flag-p27 WT or Flag-p27-T187A along with other constructs. (h) The working model for Skp2 E3 ligase-mediated cell growth, cell migration, cell cycle checkpoint, polyploidy and tumorigenesis. Skp2 interacts with mH2A1 and induces its ubiquitination and degradation. mH2A1 degradation induced by Skp2 leads to gene and protein expression of CDK8, which may serve as a kinase for p27 or regulate Cyclin A/CDK2 to drive p27 phosphorylation at T187, leading to promoting Skp2-mediated p27 ubiquitination and degradation, which may contribute to cell growth, cell migration, G2/M arrest, polyploidy and tumorigenesis. Alternatively, Skp2–mH2A1–CDK8 axis may regulate these processes independently of p27 regulation. Figure 7: CDK8 phosphorylate p27 at T187 and facilitates Skp2-mediated p27 ubiquitination and degradation. ( a ) 293T cells stably expressing luciferase shRNA (shLuc) or Skp2 shRNA (shSkp2) were transfected with the indicated plasmids and harvested for in vivo ubiquitination assay. ( b ) 293T cells stably expressing luciferase shRNA (shLuc) or CDK8 shRNA (shCDK8) were transfected with the indicated plasmids and harvested for in vivo ubiquitination assay. ( c ) 293T cells stably expressing luciferase shRNA (shLuc) or CDK8 shRNA (shCDK8) were transfected with the indicated plasmids and harvested for in vivo ubiquitination assay. ( d ) Cell lysates from 293T cells transfected with vector or CDK8 along with WT Flag-p27 or Flag-p27-187A were immunoprecipitated with Flag antibody and subjected to the immunoblotting assay. p27 phosphorylation at T187 was detected by using an antibody against phosphorylated p27 at T187. ( e ) Cell lysates from Luc or CDK8 knockdown 293T cells transfected with vector or Flag-p27 were immunoprecipitated with Flag antibody and subjected to the immunoblotting assay. p27 phosphorylation at T187 was detected by using an antibody against phosphorylated p27 at T187. ( f ) CDK8 phosphorylates p27 in vitro . Immunopurified Flag-p27 proteins were incubated with or without recombinant active CDK8 or CDK8-KD proteins and subjected to the immunoblotting assay. p27 phosphorylation at T187 was detected by using an antibody against phosphorylated p27 at T187. ( g ) In vivo ubiquitination assay of 293T cells transfected with Flag-p27 WT or Flag-p27-T187A along with other constructs. ( h ) The working model for Skp2 E3 ligase-mediated cell growth, cell migration, cell cycle checkpoint, polyploidy and tumorigenesis. Skp2 interacts with mH2A1 and induces its ubiquitination and degradation. mH2A1 degradation induced by Skp2 leads to gene and protein expression of CDK8, which may serve as a kinase for p27 or regulate Cyclin A/CDK2 to drive p27 phosphorylation at T187, leading to promoting Skp2-mediated p27 ubiquitination and degradation, which may contribute to cell growth, cell migration, G2/M arrest, polyploidy and tumorigenesis. Alternatively, Skp2–mH2A1–CDK8 axis may regulate these processes independently of p27 regulation. Full size image Notably, the ability of CDK8 to promote p27 ubiquitination was compromised on Skp2 knockdown, suggesting that CDK8 may function upstream of Skp2 to facilitate Skp2-mediated ubiquitination and degradation of p27. Indeed, we found that the ability of Skp2 to promote p27 ubiquitination was also compromised on CDK8 knockdown ( Fig. 7c ). However, CDK8 overexpression did not affect Akt ubiquitination by SCF–Skp2 ( Supplementary Fig. 7a ). These results suggest that CDK8 cooperates with Skp2 to regulate p27 ubiquitination and degradation. CDK8 not only serves as a transcription regulator, but also a protein kinase. The finding that CDK8 only regulates p27 protein expression and stability ( Supplementary Fig. 7b–d and Supplementary Fig. 8a,b ), but not p27 mRNA level ( Supplementary Fig. 7e ), suggests that CDK8 may function as a kinase for p27 and in turn regulates p27 ubiquitination and degradation. To test this hypothesis, we determined whether CDK8 interacts with p27. CO-IP assay revealed that endogenous CDK8 could interact with exogenous and endogenous p27 ( Supplementary Fig. 8c,d ). We next determined whether CDK8 phosphorylates p27 and found that CDK8 overexpression induced p27 phosphorylation at T187 residue ( Fig. 7d ), while CDK8 silencing reduced it ( Fig. 7e ). In vitro kinase assay further showed that CDK8, but not kinase dead CDK8 (CDK8-KD), could induce p27 phosphorylation at T187 ( Fig. 7f ). Phosphorylation of p27 at T187 by CDK2 is thought to be critical for Skp2-mediated p27 ubiquitination and degradation. Our finding that CDK8 is likely a kinase to phosphorylate p27 at T187 raises the possibility that CDK8 may trigger p27 phosphorylation at T187, in turn facilitating p27 ubiquitination and degradation. This was indeed a case, since CDK8 promoted ubiquitination of WT p27, but not ubiquitination of p27-T187A mutant ( Fig. 7g ). Accordingly, our results suggest that CDK8 may be a kinase for p27 and that phosphorylation of p27 at T187 induced by CDK8 is required for CDK8-mediated ubiquitination of p27. Our study has revealed several unexpected findings with important clinical implications. First, our study provides the first evidence of how mH2A1 protein abundance and stability is regulated. The exchange of the canonical H2A histones for the mH2A variant is one of the most striking epigenetic alterations at the level of the nucleosome [26] . There is an increasing interest in analysing the role of histone variant mH2A1 in cancer, but little is known about the molecular mechanism that control mH2A1 protein levels. In the present study, we unequivocally showed that Skp2 SCF is an E3 ligase for mH2A1, which triggers K48-linked ubiquitination and degradation of mH2A1. Surprisingly, while Skp2 triggers K48-linked ubiquitination of mH2A1, it also induces K63-linked ubiquitination of mH2A1 ( Fig. 2d ). Since K63-linked ubiquitination normally does not cause protein degradation, it is likely that Skp2 may also negatively regulate mH2A1 transcriptional activity through nonproteolytic K63-linked ubiquitination of mH2A1. As Skp2 expression was negatively associated with mH2A1.1 ( r= −0.624, P <0.001) and mH2A1.2 ( r= −0.578, P <0.001) in clinical samples, the deregulation of mH2A1 may represent an oncogenic event. This result also implicates that Skp2 overexpression may contribute to breast cancer pathogenesis by abolishing of mH2A1, which can alter cancer cell proliferation [27] . This notion is indeed supported by our results using animal model showing that mH2A1 silencing rescues tumour suppressive effect on Skp2 loss ( Fig. 4f ). Our data also suggest a new approach to increase mH2A1 levels by Skp2 targeting, which may have an important clinical usage for the treatment of cancer and certain diseases. For example, it is found that elevated mH2A1 expression facilitates the sensitivity of Huntington's disease to the treatment of histone deacetylase inhibitors [28] . It will be interesting to see if the combination of Skp2 inhibition by a specific Skp2 inhibitor [29] along with histone deacetylase inhibitors yields better efficacy for Huntington's disease and/or cancer. Second, we have identified the new role of mH2A1 and CDK8 in orchestrating G2/M checkpoint and polyploidy in primary MEFs. We showed that upregulation of mH2A1 or downregulation of CDK8 in primary MEFs not only regulates cell growth and migration, but also causes G2/M arrest and polyploidy, similar to Skp2 deficiency does. While exactly how polypolidy is regulated by Skp2, mH2A1 and CDK8 remains unclear, it is likely that defect in mitosis may be one of the mechanisms accounting for polyploidy as it was shown that defect in mitosis can link to polyploidy [30] . However, such assumption requires further investigation. Third, our study also provides importantly novel mechanism by which oncogenic Skp2 regulates G2/M arrest, polyploidy, cell growth, cell migration and tumorigenesis. We showed upregulation of mH2A1 that leads to the downregulation of CDK8 is responsible for these phenotypes regulated by Skp2 deficiency. While G2/M arrest and polypoloidy has impact on tumorigenesis, they are not very likely involved in Skp2–mH2A1–CDK8-mediated tumorigenicity of MDA-MB-231 cells, since G2/M arrest and polyploidy regulated by Skp2, mH2A1 and CDK8 can be seen in primary MEFs, but not in MDA-MB-231 cells where p53 is mutated. Thus, the p53 status may have great impact on the role of these proteins in G2/M arrest and polyploidy. This phenomenon is also consistent with the previous study showing that Skp2 silencing induces G2/M arrest in p53-intact, but not in p53-mutant melanoma cells [12] . Therefore, it is possible that Skp2–mH2A–CDK8 axis regulates tumorigenicity of MDA-MB-231 cells by modulating cell growth and cell migration. Recent study reveals that mH2A1 is downregulated in melanoma and lung cancers [17] , [31] . It also has been reported that CDK8 expression is upregulated in melanoma and colorectal cancers [17] , [21] . However, the expression of these two markers and their prognosis value in breast cancer remain undefined. We showed that Skp2 overexpression, mH2A1 downregulation and CDK8 overexpression are detected in advanced breast cancer and all predict poor survival outcome for breast cancer patients. Our study demonstrates that the expression of mH2A1 and CDK8 in protein expression level can predict the survival outcome of breast cancer patients. Importantly, Skp2 expression positively correlated with CDK8 expression, but inversely associates with mH2A1 expression. It suggests that mH2A1 is a novel tumour suppressor, while CDK8 can serve as an oncogene in breast cancer. Finally, our study reveals that CDK8 may be a kinase for p27. CDK8 is shown to drive phosphorylation of p27 at T187 residue, facilitating Skp2-mediated p27 ubiquitination and degradation. Previous studies reveal that Cyclin E/CDK2 or Cyclin A/CDK2 is also a kinase for T187 phosphorylation of p27. While CDK8 may serve as a direct kinase for p27 and trigger T187 phophorylation, it may also regulate p27 T187 phosphorylation indirectly through modulating Cyclin A/CDK2 activity [32] , [33] . In support of this notion, we found that CDK8 knockdown in breast cancer cells reduces Cyclin A, but not CDK2 and Cyclin E, protein expression, accompanied by a reduction in pRb phosphorylation, a readout for CDK2 kinase activity ( Supplementary Fig. 5c ). Thus, our results suggest that CDK8 may regulate p27 T187 phosphorylation and degradation by either serving as a kinase for p27 or regulating Cyclin A/CDK2 kinase activity. Notably, we show that CDK8 and Skp2 functionally rely on each other to regulate ubiquitination and degradation of p27. The rationalized model to explain this phenomenon is that CDK8 firstly regulates p27 phosphorylation at T187, which may provide a priming site for Skp2 and allow Skp2 to promote ubiquitination and degradation of p27. Given that Skp2 is a positive regulator for CDK8 gene expression, it is likely that Skp2 may also orchestrate p27 T187 phosphorylation by upregulating CDK8 expression, thereby providing a positive feedback loop to further facilitate p27 ubiquitination and degradation. As previous studies reveal that p27 is an important Skp2 downstream substrate that mediates Skp2’s biological functions [10] , [34] , it is very likely that CDK8 may converge on the p27 pathway to regulate Skp2-mediated cell cycle progression, polyploidy and tumorigenesis. In summary, our study uncovers a molecular mechanism controlling mH2A1 stability and identifies the Skp2–mH2A1–CDK8 axis as a key pathway for regulating G2/M transition, polyploidy, cell proliferation, cell migration and breast cancer development ( Fig. 7h ). We also show that CDK8 promotes phosphorylation of p27 at T187 and then induces p27 ubiquitination and degradation in a Skp2-dependent manner. Given that Skp2 and CDK8 are overexpressed in breast cancer and their overexpression promotes breast cancer development in mouse models, pharmacological inactivation of Skp2 and CDK8 is therefore a potential strategy for those cancers with Skp2 and CDK8 overexpression. Cell lines and reagents MEFs from Skp2 +/+ and Skp2 −/− mice were prepared as previously described [19] . 293T cells, MDA-MB-231 and BT474 were obtained from American Type Culture Collection and cultured in DMEM medium containing 10% foetal bovine serum (FBS). Flag–Skp2 and Flag-ΔN-Skp2 (amino acids 91–424) were described [20] . mH2A1.1, mH2A1.2 and pLPC-mH2A1.1-mCherry plasmids were gifted from Dr E. Bernstein. The mH2A1.1-mCherry constructs expressing various fragments of mH2A1.1 were generated from the retroviral construct pLPC-mH2A1.1-mCherry by using a PCR-based gene deletion strategy based on the domain structure of mH2A1.1. dC, deletion of the macro domain; dL, deletion of the linker domain; and dN, deletion of the H2A domain. CDK8 and CDK8-KD expressing plasmid were obtained from Dr J.Y. Ji. Western blotting Western blotting was performed as previously described [20] . The following antibodies were used for IP or immunoblotting (IB): Skp2 antibody (IP: 1:200, IB: 1:2,000, Invitrogen-323300), mH2A1 (IP: 1:200, IB: 1:2,000, Millipore 07-219), CDK8 (IB: 1:1,000, Santa Cruz-1521), Flag antibody (M2) (IP: 1:100; IB: 1:1,000, Sigma-F1804), Xpress antibody (IP:1:200; IB: 1:3,000, Invitrogen R910-25), DsRed antibody (IB, 1:1,000, Clontech 632496), P27 antibody (IP, 1:100; IB, 1:1,000; BD Transduction Lab-610241), Cyclin A antibody (IB, 1:2,000, Santa Cruz-751), Cyclin E antibody (IB, 1:2,000, Santa Cruz-481), CDK2 antibody: (IB, 1:2,000, Cell signaling-2546P) and β-actin antibody (IB: 1:3,000, Sigma A1978). Full images of IBs are shown in Supplementary Figs 9–17 . Mass spectrometry and protein identification 293T cells stably transfected with vector or Xpress-Skp2 (XP-Skp2) were lysed in E1A buffer (250 mM NaCl, 50 mM HEPES pH 7.5, 0.1% Nonidet P40 and 5 mM EDTA), and 8 mg of protein lysates were immunoprecipitated with Xpress antibody, which is not coupled to other matrix, washed by E1A buffer, and subjected to SDS–PAGE. Protein bands were excised from silver-stained gels, and destained by SilverQuest (Invitrogen) and dried in a SpeedVac concentrator. The gel pieces were then swollen in 30 μl of 20 mM ammonium bicarbonate buffer containing 0.01 mg ml −1 modified sequencing grade trypsin (Promega) and incubated overnight at 37 °C. The resulting peptides were extracted sequentially with 1% TFA and 0.1% TFA/60% ACN and the combined extracts lyophilized and analysed using a Qstar XL Q-TOF mass spectrometer (Applied Biosystems) coupled to an UltiMate Nano LC system (Dionex/LC Packings, Amsterdam, Netherlands). Proteins were identified by MASCOT software (Matrix Science, Boston, MA) against the NCBI protein database. The following search parameters were used: trypsin was used as the digestive enzyme, mass tolerance for monoisotopic peptide window was set to ±1.0 Da, the MS/MS tolerance window was set to ±0.5 Da, one missed cleavage was allowed, and carbamidomethyl, deamidated and oxidized methionine were chosen as variable modifications. The utilized matching criteria were as follows: each identified peptide had to score >20, and at least two unique peptides had to be specific to the identified protein. Ubiquitination assay in vitro and in vivo In vivo ubiquitination assays were performed as described [35] . In brief, 293T cells were transfected with the indicated plasmids for 48 h and lysed by the denatured buffer (6 M guanidine-HCl, 0.1 M Na2HPO4/NaH2PO4, 10 mM imidazole). The supernatants were incubated with nickel beads for 3 h, washed and subjected to IB analysis. For in vitro ubiquitination assays, Flag–Skp2 and Flag–mH2A1 proteins purified from the 293T cells were incubated with for at 37 °C for 3 h in 20 ml of reaction buffer (20 mM HEPES (pH 7.4), 10 mM MgCl2, 1 mM DTT, 59 mM ubiquitin, 50 nM E1, 850 nM of Ubc13/Uev1a, 1 mM ATP, 30 mM creatine phosphate and 1 U of creatine kinase). Proteins were eluted in SDS-sample buffer and immunoblotted with anti-mH2A1 antibody. GST pull-down assays For in vitro GST–Skp2 and mH2A1 interaction, GST–Skp2 proteins were purified from the bacterial lysates of BL21 competent cells using the glutathione-agarose beads according to the manufacturer’s standard procedures. The GST–Skp2 proteins bound to glutathione beads were then incubated with the in vitro translated Flag–mH2A1 at 4 °C overnight in the interaction buffer (20 mM HEPES, PH 7.9, 150 mM KCl. 5 mM EDTA, 0.5 mM DTT, 0.1% (v/v) Nonidet p40, 0.1% (w/v) BSA, 1 mM PMSF, and 10% Glycerol), washed by the NETN buffer (20 mM Tris, pH 8.0, 100 mM NaCl, 6 mM MgCl2, 1 mM EDTA, 0.5% Nonidet P40, 1 mM DTT, 8% glycerol, 1 mM PMSF) four times, and subjected to 8% SDS–PAGE, followed by IB. MTT cell growth assay and cell migration assay For MTT (3-(4,5-Dimethylthiazol-2-yl)-2,5-diphenyltetrazolium Bromide) cell growth assay, cells were planted in 96-well plates with a concentration of 1,000 cells per well. About 20 μl of 5 mg ml −1 MTT was added into the media and cultured for 4 h. Then the media were removed, DMSO was added to dissolve the deposits. At last, the absorbance at 550 nm can be measured by the microplate reader. Cell migration assay was carried out in 24-well transwell plate with 8-μm polyethylene terephalate membrane filters (Falcon cell culture insert (Becton Dickinson)) separating the lower and upper culture chambers. In brief, ~1 × 10 5 cells were seeded into in the upper chamber with serum-free DMEM medium. The bottom chamber contained DMEM with 10% FBS. After the incubation period, the filter was removed and non-migrant cells on the upper side of the filter were detached using a cotton swab. Cells that migrated to the lower side of the membrane were stained with 0.1% crystal violet for 20 min and counted from three random fields. Flow cytometry For DNA content studies, cells were harvested, washed with phosphate-buffered saline and fixed in ice-cold 70% ethanol. Cells were then stained with 0.01% propidium iodide solution for 30 min. The ethanol was removed by spinning down for 5 min, and cells were analysed with a FACSCan flow cytometer. Viral infection For retroviral infection, retroviral plasmids were transfected into Phoenix packing cells for 2 days, and then the virus-containing medium was harvested to infect target cells. For lentiviral short hairpin RNA (shRNA) infection, 293T cells were co-transfected with shRNA against Luc, Skp2 or mH2A1 along with packing plasmids (deltaVPR8.9) and envelope plasmid (VSV-G) using the calcium phosphate precipitation method. Then virus particles containing Skp2 and green fluorescent protein shRNAs were used to infect mammalian cells after 2 days. All the infected cells were cultured in the medium containing 2 μg ml −1 puromycin for 1 week. The following lentiviral shRNAs were used for transfection: Skp2-lentiviral shRNA-1 (5′- GATAGTGTCATGCTAAAGAAT -3′), Skp2-lentiviral shRNA-2 (5′- GCCTAAGCTAAATCGAGAGAA -3′) and mH2A1-lentiviral shRNAs, as previously described [17] , which were obtained from Dr E. Bernstein. In vitro kinase assay CDK8-WT and CDK8-KD proteins were synthesized in vitro using the TNT High-Yield Protein Expression System (Promega). Flag-p27 was obtained by IP using anti–Flag agarose from the lysates of 293 cells overexpressing Flag-p27. Then, the samples were incubated with 3 μg of CDK8-WT and CDK8-KD in 50 μl of kinase buffer (Cell Signaling Technology) containing 10 μM ATP at 30 °C for 30 min. Subsequently, the samples were subjected to SDS–PAGE, followed by IB. Microarray analysis WT and Skp2 −/− LT-HSCs (long-term haematopoietic stem cells) were isolated from WT and Skp2 −/− mice as described [36] . Total RNAs from WT and Skp2 −/− LT-HSCs were subjected to microarray analysis. Microarray experiments were carried out using the ‘Human Whole Genome Oligo Microarray Kit’ from Agilent (Agilent Technologies, Alto, CA) and the manufacturer’s protocol was followed. Detailed protocol can be found at Agilent website: www.Agilent.com . Briefly, 200 ng of total RNA from each sample was used and labelled with either Cy3- or Cy5-CTP and after 17 h hybridization at 65 °C, the arrays were washed and scanned with Agilent’s dual-laser based scanner. Then, Feature Extraction software GE2-v5_95 was used to link a feature to a design file and determine the relative fluorescence intensity between the two samples. Gene lists were created using P value information from the internal replicates within the microarray. The result was shown as a ratio between Skp2 −/− and WT HSCs ( Skp2 −/− versus WT ). In vivo tumorigenesis assay For in vivo tumorigenesis assays, MDA-MB-231 stable cells mixed with matrigel (1:1) were subcutaneously injected into the left flank of 6-week-old female nude mice. Tumour size was measured weekly using a caliper, and the tumour volume was determined with the standard formula: L × W 2 × 0.52, where L is the longest diameter and W is the shortest diameter. The animal study was approved by the Institutional Animal Care and Use Committee (IACUC) from MD Anderson Cancer Center. Patients and human materials The institutional review board of Chi-Mei Medical Center had approved the study by using formalin-fixed tissue from BioBank (IRB9812-012). As a rule set by MOHW (Taiwan), informed consent had been obtained for every case enroled in the BioBank. IHC analysis was performed on 189 consecutively treated breast carcinoma patients who underwent modified radical mastectomy between 1997 and 2003. No adjuvant chemotherapy was given in these patients. Pathological staging was assigned based on the 7th edition of American Joint Committee on Cancer (AJCC) system. IHC and scoring The procedures of IHC studies were performed as previously described (Cell. 2012 May 25;149(5):1098-111.). In brief, sections were cut on an adhesive-coated glass slides at 3-μm thickness. For staining in human samples, the slides were incubated with primary antibodies against Skp2 (Invitrogen, 1:100), mH2A1.1 (Cell signaling, 1:50), mH2A1.2 (1:100), CDK8 (Santa Cruz, 1:100), polyclonal cleaved caspase-3 (Cell Signaling, 1:100) and Ki-67 antibody (Epitomics, 1:160). Primary antibodies were detected using the ChemMateDAKO EnVision kit (DAKO, K5001). The slides were incubated with the secondary antibody for 30 min and developed with 3,3'-diaminobenzidine for 5 min. Incubation without the primary antibody was used as a negative control. Immunoexpression of cleaved caspase-3 was scored by two experienced pathologists using a multiheaded microscope to reach a consensus for each case. The staining was evaluated based on a combination of both the percentage and intensity of positively stained tumor cells to generate an H -score, which was calculated using the following equation: H -score=Σ P i ( i +1), where i is the intensity of the stained tumor cells (0 to 4 +), and P i is the percentage of stained tumor cells for each intensity. The final score=extent score × intensity score: −=negative immunostaining: score 0–2;+=moderate immunostaining; score 3–5; ++=strong immunostaining; score=>6. To evaluate the stained sections descriptively with Ki-67 antibodies, the number of positive cells was counted. Cell nuclei for Ki-67 with bright brown colour were considered as positive cells. Cell counts were made at × 40 magnification with conventional light microscope in 10 randomly selected fields, counting a minimum of 1,000 cells. Labelling Index (LI)=number of IHC positive cells × 100/total number of cells observed. Statistical analysis Statistical analyses were performed using the SPSS 14 software package. The Kruskal–Wallis H -test and Mann–Whitney U -test were used to assess the differential expression level of Skp2, mH2A1.1, mH2A1.2 and CDK8 expression in relation to important clinicopathologic variables. The Pearson’s correlation coefficient was used to clarify the association between Skp2, mH2A1.1, mH2A1.2 and CDK8 expression levels. The endpoint analysed was DSS and distal MeFS, calculated from the starting date of surgery to the date disease-related death or metastatic events occured. The median period of follow-up was 107 months (range, 6 to 144). Univariate survival analysis was performed using the Cox proportional hazards model. Survival curves were plotted using the Kaplan–Meier method, and log-rank tests were performed to evaluate prognostic differences between groups for categorical variables. A multivariate model was performed using Cox proportional hazards regression, including parameters with univariate P <0.05. Since primary tumour status (pT) and nodal status (pN) are component factors of tumour stage, only stage was enroled into multivariate analysis. For all analyses, two-sided tests of significance were used with P ≤ 0.05 considered significant. Accession codes : Gene Expression Omnibus. The data were deposited to Gene Expression Omnibus (GEO), the record number is GSE23064; Link: http://www.ncbi.nlm.nih.gov/geo/query/acc.cgi?token=hfinxomsugyialo&acc=GSE23064 How to cite this article: Xu, D. et al . Skp2–MacroH2A1–CDK8 axis orchestrates G2/M transition and tumorigenesis. Nat. Commun. 6:6641 doi: 10.1038/ncomms7641 (2015).